p53 increases MHC class I expression by upregulating the endoplasmic reticulum aminopeptidase ERAP1 The p53 tumour suppressor has an important role in cancer cells. Here we show that p53 regulates expression of major histocompatibility complex I on the cell surface. We show that the tumour cell line HCT116, which lacks p53 exhibits significantly lower major histocompatibility complex I expression than its wild-type counterpart. Using a combination of chromatin immunoprecipitation sequencing and gene expression analysis, we demonstrate that p53 upregulates expression of endoplasmic reticulum aminopeptidase 1 by binding to its cognate response element in the ERAP1 gene. Silencing of p53 decreases endoplasmic reticulum aminopeptidase 1 protein levels and therefore major histocompatibility complex I expression. We further show that this mechanism operates in A549 cells infected with H1N1 influenza virus, in which H1N1 activates p53, leading to endoplasmic reticulum aminopeptidase 1 upregulation and a corresponding increase in major histocompatibility complex I expression. Our study suggests a previously unrecognized link between p53 function and the immunosurveillance of cancer and infection. The tumour suppressor protein p53 regulates diverse cellular processes including apoptosis, cell cycle, senescence and metabolism [1] . It does so by sensing cellular and genotoxic stress signals and responds by activating or repressing gene targets that bear a p53-response element (p53RE) in their regulatory region. Recent evidence suggests that p53 participates in a broader range of cellular activities than previously thought [2] , including, perhaps, the immune response [3] , [4] . We had observed that in p53 isogenic HCT116 cell lines, differing only in their p53 status, major histocompatibility complex (MHC) Class I expression at the cell surface was also disparate, and wondered whether this observation might strengthen the evidence between p53 and regulation of immune responses. Appropriate regulation of MHC expression is important for effective tumour surveillance and protection against viral infection [5] , [6] , but no interaction of p53 and the MHC I pathway had yet been convincingly shown. The MHC class I antigen presentation pathway comprises a series of complex steps, which integrate degradation and preparation of the peptides to be loaded for presentation with the assembly and expression of the MHC molecules themselves. Regulation of MHC I expression thus occurs at multiple levels and involves numerous components of the presentation pathway machinery [7] . One molecule that has received much interest is the endoplasmic reticulum aminopeptidase 1 ( ERAP1 ), which is responsible for the final trimming of antigen precursors before loading into MHC class I proteins [8] . Defects in ERAP1 result in changes in MHC class I expression and impaired T-cell responses [9] , and ERAP1 allelic variants are associated with diseases including ankylosing spondylitis and hypertension [10] , [11] , [12] . Altered ERAP1 expression was also observed in some human cancer cell lines [13] , [14] and has recently been linked to clinical outcome in cervical carcinoma [15] . In this study, we asked how the p53 status of cells relates to their MHC I expression. Using two isogenic human colon carcinoma cell lines HCT116 ( p53 −/− and p53 +/+ ), we show that p53 can affect MHC I levels via transcriptional regulation of ERAP1. We use expression profiling analysis to identify p53-regulated genes in these cells and validate ERAP1 as a direct target of p53. This mechanism is also active during viral infection, as in a human pulmonary epithelial cell line exposed to H1N1 influenza virus, p53 is activated and in turn increases the surface expression of MHC class I via ERAP1. Our data reveal an important new role for p53 in the immune response and define a mechanism that explains the relationship between p53 and MHC I in both transformed and virally infected cells. MHC class I levels are higher in p53 +/+ than p53 −/− cells We used a pair of isogenic cell lines that differ in their p53 status (HCT116 p53 +/+ and HCT116 p53 −/− ), and assessed the levels of MHC I on their cell surface. HCT116 ( p53 +/+ ) cells expressed substantially more surface MHC Class I molecules than p53 −/− cells, evident by flow cytometry ( Fig. 1a ), and fluorescence microscopy ( Fig. 1b ). The same results were observed in two osteosarcoma cell lines that similarly differ in p53 expression, U2OS ( p53 +/+ ) and Saos-2 ( p53 −/− ), with higher MHC class I expression in the U2OS cells, which possess wild-type p53 alleles ( Fig. 1c,d ). Thus, we hypothesized that the differential expression of MHC Class I observed might be linked to the differential p53 status of the cell lines tested. The effect of p53 expression was specific for MHC I, and did not affect MHC II levels ( Fig. 1a,c ). 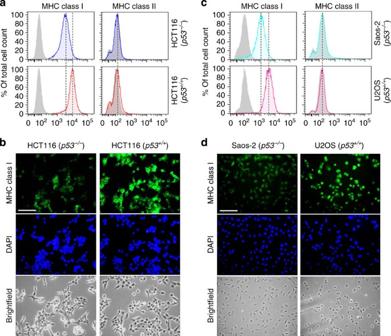Figure 1: MHC class I is differentially expressed inp53+/+andp53−/−cell lines. (a) Flow cytometric analysis of MHC class I (HLA-ABC, W6/32 labelling) and MHC class II (HLA-DR, L243 labelling) expression on HCT116 (p53+/+) (red) and HCT116 (p53−/−) (blue) cells. Cells incubated with fluorescence-labelled secondary antibodies alone served as background controls (Grey). (b) Immunofluorescence images of MHC class I expression shown by W6/32 labelling of HCT116 (p53+/+) and HCT116 (p53−/−) cells. DAPI and Brightfield images confirm the relatively equal number of cells captured. Scale bar, 50 μm. (c) Flow cytometric analysis of MHC class I (W6/32 labelling) and MHC class II (L243 labelling) expression in U2OS (p53+/+) (magenta) and Saos-2 (p53−/−) (cyan) cells. (d) Immunofluorescence images of MHC class I expression shown by W6/32 labelling of U2OS (p53+/+) and Saos-2 (p53−/−) cells. Scale bar, 50 μm. Figure 1: MHC class I is differentially expressed in p53 +/+ and p53 −/− cell lines. ( a ) Flow cytometric analysis of MHC class I (HLA-ABC, W6/32 labelling) and MHC class II (HLA-DR, L243 labelling) expression on HCT116 ( p53 +/+ ) (red) and HCT116 ( p53 −/− ) (blue) cells. Cells incubated with fluorescence-labelled secondary antibodies alone served as background controls (Grey). ( b ) Immunofluorescence images of MHC class I expression shown by W6/32 labelling of HCT116 ( p53 +/+ ) and HCT116 ( p53 −/− ) cells. DAPI and Brightfield images confirm the relatively equal number of cells captured. Scale bar, 50 μm. ( c ) Flow cytometric analysis of MHC class I (W6/32 labelling) and MHC class II (L243 labelling) expression in U2OS ( p53 +/+ ) (magenta) and Saos-2 ( p53 −/− ) (cyan) cells. ( d ) Immunofluorescence images of MHC class I expression shown by W6/32 labelling of U2OS ( p53 +/+ ) and Saos-2 ( p53 −/− ) cells. Scale bar, 50 μm. Full size image ERAP1 is a potential p53-target gene To understand how p53 expression and MHC I levels might be linked, we asked whether the expression of any other molecules in the MHC I presentation pathway were also affected by p53 expression. We transfected HCT116 ( p53 −/− ) with constructs encoding either wild-type p53, or one of six mutant p53 sequences, then subjected the cells to microarray analysis of global gene expression. The dominant-negative effects of the six mutant p53 constructs used were previously reported (IARC p53 database) and again confirmed by a correlation analysis ( R 2 ) of our customized luciferase assays using 16 dinucleotide core combinations [16] ( Supplementary Fig. S1a–f ) and a ProLabel Protein–DNA binding assay using p53RE of p21 gene in p53 −/− HCT116 cells ( Supplementary Fig. S1g ). Fold change analysis of gene expression was applied to genes involved in four key stages of the MHC class I presentation pathway: (i) protein breakdown ( PSMB10 / MECL1 , PSMB8 / LMP7 , PSMB9 / LMP2 , PSME1 / PA28α and PSME2 / PA28β ); (ii) peptide transport ( TAP1 , TAP2 , TAPBP , TAPBPL , HSPA5 / BIP , CALR , CALR3 and CANX ); (iii) peptide trimming ( ERAP1 and ERAP2 ); and (iv) MHC class I structures ( HLA-B and B2M ). The heatmap representation of these data ( Fig. 2a ) shows that TAP1 and ERAP1 are two potential p53 targets, both exhibiting greater than 0.5-fold increase in expression in response to transfection of wild-type, but not mutant, p53. To confirm the microarray data, we performed real-time qPCR analysis using the isogenic p53 +/+ and p53 −/− HCT116 cells treated with Nutlin 3, an mdm2-antagonist that specifically blocks p53-mdm2 interactions and rapidly induces endogenous p53 protein accumulation. The results correlated well with the microarray data; mRNA levels of both TAP1 and ERAP1 were markedly increased in Nutlin 3-treated cells, in a p53-dependent manner, while other genes showed little response to Nutlin 3 ( Fig. 2b ). As the regulation of TAP1 by p53 has been previously reported [17] , we shall focus here on the relationship between p53 and ERAP1 . 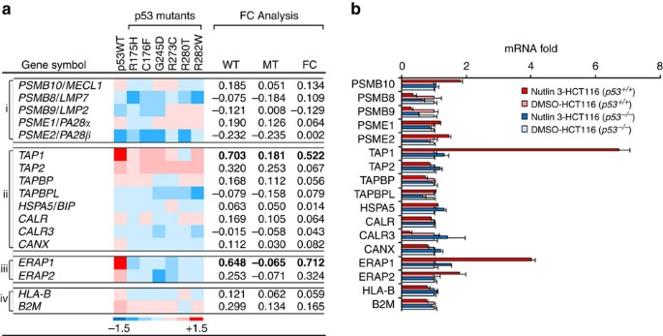Figure 2: Regulation of genes involved in the MHC class I presentation pathway by p53. (a) Heatmap representation of Exon array data shows the fold change in mRNA level of genes involved in the MHC class I presentation pathway, grouped according to function: (i) protein breakdown; (ii) peptide transport; (iii) peptide trimming; and (iv) MHC class I structures. The normalized fold change (FC) for each gene was calculated by the difference between the fold change in p53WT (WT) transfected cells and the average fold change in six loss-of-function p53 mutants (MT)-transfected cells in relative to pcDNA3.1 control-transfected cells. (b) Real-time qPCR analysis of mRNA expression of MHC presentation pathway genes in Nutlin 3-treated HCT116 (p53+/+) and HCT116 (p53−/−) cells. Data are representative of three independent experiments (mean±s.d.) and presented as fold change in mRNA expression in Nutlin 3-treated relative to DMSO-treated (control) cells, normalized toHPRTgene expression. Figure 2: Regulation of genes involved in the MHC class I presentation pathway by p53. ( a ) Heatmap representation of Exon array data shows the fold change in mRNA level of genes involved in the MHC class I presentation pathway, grouped according to function: (i) protein breakdown; (ii) peptide transport; (iii) peptide trimming; and (iv) MHC class I structures. The normalized fold change (FC) for each gene was calculated by the difference between the fold change in p53WT (WT) transfected cells and the average fold change in six loss-of-function p53 mutants (MT)-transfected cells in relative to pcDNA3.1 control-transfected cells. ( b ) Real-time qPCR analysis of mRNA expression of MHC presentation pathway genes in Nutlin 3-treated HCT116 ( p53 +/+ ) and HCT116 ( p53 −/− ) cells. Data are representative of three independent experiments (mean±s.d.) and presented as fold change in mRNA expression in Nutlin 3-treated relative to DMSO-treated (control) cells, normalized to HPRT gene expression. Full size image The ERAP1 gene contains a functional p53RE Having identified ERAP1 as a potential target of p53, we next wanted to ask whether p53 was directly or indirectly regulating ERAP1 expression. We first validated the microarray ERAP1 expression data by real-time qPCR analysis. This confirmed that increasing ERAP1 mRNA expression was restricted to cells overexpressing wild-type p53, and not affected by overexpression of any of the mutant forms of p53 tested ( Fig. 3a ). Basal expression of ERAP1 mRNA was also measured by real-time qPCR and was at least threefold higher in p53 +/+ than p53 −/− HCT116 cells ( Fig. 3b ). This was also observed at the protein level ( Fig. 3c ). Although ERAP2 had been weakly activated by wild-type p53 according to the microarray data ( Fig. 2a ), we did not observe any difference in the basal level of protein expression between the p53 +/+ and p53 −/− HCT116 cell lines ( Fig. 3c ), and therefore did not pursue these findings further. To understand how ERAP1 expression was regulated by p53, we asked whether ERAP1 contained any possible p53REs that would allow a direct interaction. We employed Chromatin immunoprecipitation (ChIP)-coupled sequencing (ChIP-seq), which facilitates identification of binding sequences within the target gene and provides evidence for direct interactions between proteins and those specific DNA sequences. As cancer cell lines can harbour multiple undefined genetic aberrations, we used normal healthy human PBMCs to ensure robust genome-wide coverage. ChIP-seq peaks indicating two potential p53REs that conform to the classical RE motifs [18] were identified in the intronic region of ERAP1 genes ( Fig. 3d ). The putative RE sequences were then cloned upstream of the SV40 minimal promoter into a pGL3-promoter vector and co-transfected with either p53WT or mutant constructs, into HCT116 p53 −/− cells. Luciferase assays were performed to establish sensitivity of the potential REs to p53. As a positive control, the luciferase construct containing the p53RE from p21 was used, and was indeed sensitive to p53WT but not the R175H mutant. The p53WT construct activated luciferase gene expression in ERAP1 constructs containing the putative RE2 but not RE1, while the R175H mutant failed to activate luciferase expression in cells containing either of the putative RE constructs ( Fig. 3d ). The ERAP1-RE2 sequence also bound strongly to p53WT protein compared with the weak affinity to the six loss-of-function p53 mutants ( Fig. 3e ) and thus is a bona fide p53RE. Finally, RE2 was mapped to the identified ChIP-seq peak as well as the genomic region of ERAP1 ( Fig. 3f ). In summary, we showed here that ERAP1 levels are affected by p53 expression and this likely occurs due to a direct interaction of the p53 protein with the identified RE sequence in the ERAP1 gene. 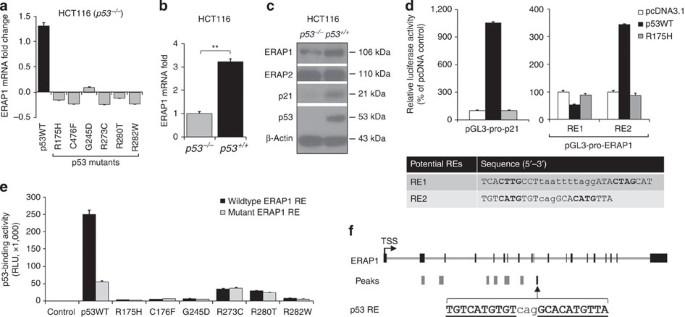Figure 3: ERAP1 is transcriptionally regulated by p53 via abona fidep53RE. (a) Real-time qPCR validation of fold change in ERAP1 mRNA expression in HCT116 (p53−/−) cells transfected with wild-type p53 (p53WT) or one of 6 p53 mutants, compared with cells transfected with the pcDNA3.1 control. (b) Real-time qPCR analysis of relative basal ERAP1 mRNA expression levels inp53+/+andp53−/−HCT116 cells. **P<0.01 (two-tailed Student’st-test). (c) Western blot of ERAP1, ERAP2, p21, p53 and β-actin (loading control) in HCT116 (p53+/+) and HCT116 (p53−/−) cells. (d) Dual-luciferase assay results of p53WT or the p53 dominant-negative mutant R175H co-transfected with different ERAP1 RE constructs (pGL3-pro-ERAP1-RE1 and RE2, sequences listed in the table at the bottom panel) into HCT116 (p53−/−) cells. Data are presented as percentage luciferase activity relative to the pcDNA3.1 control vector-transfected cells. Luciferase assay using p21 promoter construct (pGL3-pro-p21) serves as the positive control. (e) Binding affinity of wild-type p53 (p53WT) or the six p53 mutants to the identified ERAP1 p53RE sequences (wild-type or mutant) was determined by ProLabel Protein–DNA binding assay. (f) Schematic representation of identifiedERAP1p53RE (RE2) in relation to the ChIP-seq peaks and genomic localization ofERAP1gene. TSS: transcription start site. Data are representative of three independent experiments and error bars represent s.d. of technical replicates (mean±s.d.),n=3, ina,b,d,e. Figure 3: ERAP1 is transcriptionally regulated by p53 via a bona fide p53RE. ( a ) Real-time qPCR validation of fold change in ERAP1 mRNA expression in HCT116 ( p53 −/− ) cells transfected with wild-type p53 (p53WT) or one of 6 p53 mutants, compared with cells transfected with the pcDNA3.1 control. ( b ) Real-time qPCR analysis of relative basal ERAP1 mRNA expression levels in p53 +/+ and p53 −/− HCT116 cells. ** P <0.01 (two-tailed Student’s t -test). ( c ) Western blot of ERAP1, ERAP2, p21, p53 and β-actin (loading control) in HCT116 ( p53 +/+ ) and HCT116 ( p53 −/− ) cells. ( d ) Dual-luciferase assay results of p53WT or the p53 dominant-negative mutant R175H co-transfected with different ERAP1 RE constructs (pGL3-pro-ERAP1-RE1 and RE2, sequences listed in the table at the bottom panel) into HCT116 ( p53 −/− ) cells. Data are presented as percentage luciferase activity relative to the pcDNA3.1 control vector-transfected cells. Luciferase assay using p21 promoter construct (pGL3-pro-p21) serves as the positive control. ( e ) Binding affinity of wild-type p53 (p53WT) or the six p53 mutants to the identified ERAP1 p53RE sequences (wild-type or mutant) was determined by ProLabel Protein–DNA binding assay. ( f ) Schematic representation of identified ERAP1 p53RE (RE2) in relation to the ChIP-seq peaks and genomic localization of ERAP1 gene. TSS: transcription start site. Data are representative of three independent experiments and error bars represent s.d. of technical replicates (mean±s.d. ), n =3, in a , b , d , e . Full size image Nutlin 3 increases MHC class I expression in p53 +/+ cells As shown in Figs 2b and 4a , ERAP1 mRNA expression is significantly ( P <0.01; two-tailed Student's t -test) increased in response to Nutlin 3 treatment in HCT116 ( p53 +/+ ) but not HCT116 ( p53 −/− ) cells, leading us to hypothesize that MHC class I surface expression would in turn be affected by p53-modulating agents, such as Nutlin 3, in a p53-dependent manner. To first confirm the ERAP1 mRNA data, the amount of ERAP1 protein was visualized by immunoblotting using cell lysates of Nutlin 3-treated HCT116 p53 +/+ and p53 −/− cells. Nutlin 3 treatment caused a marked increase in ERAP1 protein in HCT116 ( p53 +/+ ) cells, with concomitant p53 protein accumulation and p21 induction, while in HCT116 ( p53 −/− ) cells, there was no change in ERAP1 protein level ( Fig. 4b ). Nutlin 3-treated HCT116 ( p53 +/+ ) and HCT116 ( p53 −/− ) cells were then subjected to flow cytometric analysis of MHC class I surface expression after 24 and 48 h incubation. Increased MHC I expression was evident in p53 +/+ HCT116 cells at both time points, while no increase was seen in p53 −/− cells ( Fig. 4c ). HCT116 ( p53 −/− and p53 +/+ ) cells after 48 h of Nutlin 3 treatment were also labelled with antibodies against MHC I for fluorescence microscopic analysis ( Fig. 4d ), further demonstrating the p53-dependent increase in MHC class I expression. Genotoxic drugs also induce p53 expression, and treatment of the isogenic HCT116 cell lines with 5-fluorouracil (5-FU) accordingly increased ERAP1 mRNA expression ( Fig. 4e ) with concomitant MHC class I upregulation in p53 +/+ HCT116 cells ( Fig. 4f ). These observations were not restricted to the two cell lines tested, and similar results were obtained using the paired osteosarcoma cell lines U2OS ( p53 +/+ ) and Saos-2 ( p53 −/− ) ( Supplementary Fig. S2 ). 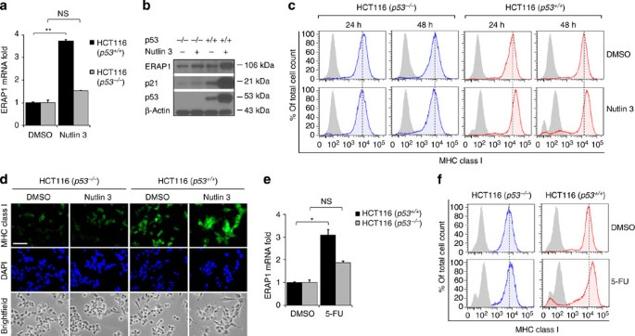Figure 4: Nutlin 3 and 5-FU treatment increases MHC class I expression in a p53-dependent manner. (a) Real-time qPCR analysis of ERAP1 mRNA expression in Nutlin 3 (25 μM) or DMSO control-treated HCT116 (p53+/+) and HCT116 (p53−/−) cells. **P<0.01, NS, not significant (two-tailed Student’st-test). (b) Western blot of ERAP1, p53, p21 and β-actin (loading control) expression in Nutlin 3 or DMSO control-treated HCT116 (p53+/+) and HCT116 (p53−/−) cells. (c) Flow cytometric analysis of MHC class I (W6/32 labelling) expression in Nutlin 3 or DMSO control-treated HCT116 (p53+/+) (Red) and HCT116 (p53−/−) (Blue) cells after 24 and 48 h treatment. Cells incubated with fluorescence-labelled secondary antibodies alone served as background controls (Grey). (d) Immunofluorescence images of MHC class I expression, shown by W6/32 labelling, of Nutlin 3 or DMSO control-treated HCT116 (p53+/+) and HCT116 (p53−/−) cells at 48 h post treatment. DAPI and Brightfield images confirm the relatively equal number of cells captured. Scale bar, 50 μm. (e) Real-time qPCR analysis of ERAP1 mRNA expression in 5-FU (50 μg ml−1) or DMSO control-treated HCT116 (p53+/+) and HCT116 (p53−/−) cells. *P<0.05, NS, not significant (two-tailed Student’st-test). (f) Flow cytometric analysis of MHC class I (W6/32 labelling) expression in 5-FU or DMSO control-treated HCT116 (p53+/+) (red) and HCT116 (p53−/−) (blue) cells at 48 h post treatment. Data are representative of three independent experiments and error bars represent s.d. of technical replicates (mean±s.d.),n=3, ina,e. Figure 4: Nutlin 3 and 5-FU treatment increases MHC class I expression in a p53-dependent manner. ( a ) Real-time qPCR analysis of ERAP1 mRNA expression in Nutlin 3 (25 μM) or DMSO control-treated HCT116 ( p53 +/+ ) and HCT116 ( p53 −/− ) cells. ** P <0.01, NS, not significant (two-tailed Student’s t -test). ( b ) Western blot of ERAP1, p53, p21 and β-actin (loading control) expression in Nutlin 3 or DMSO control-treated HCT116 ( p53 +/+ ) and HCT116 ( p53 −/− ) cells. ( c ) Flow cytometric analysis of MHC class I (W6/32 labelling) expression in Nutlin 3 or DMSO control-treated HCT116 ( p53 +/+ ) (Red) and HCT116 ( p53 −/− ) (Blue) cells after 24 and 48 h treatment. Cells incubated with fluorescence-labelled secondary antibodies alone served as background controls (Grey). ( d ) Immunofluorescence images of MHC class I expression, shown by W6/32 labelling, of Nutlin 3 or DMSO control-treated HCT116 ( p53 +/+ ) and HCT116 ( p53 −/− ) cells at 48 h post treatment. DAPI and Brightfield images confirm the relatively equal number of cells captured. Scale bar, 50 μm. ( e ) Real-time qPCR analysis of ERAP1 mRNA expression in 5-FU (50 μg ml −1 ) or DMSO control-treated HCT116 ( p53 +/+ ) and HCT116 ( p53 −/− ) cells. * P <0.05, NS, not significant (two-tailed Student’s t -test). ( f ) Flow cytometric analysis of MHC class I (W6/32 labelling) expression in 5-FU or DMSO control-treated HCT116 ( p53 +/+ ) (red) and HCT116 ( p53 −/− ) (blue) cells at 48 h post treatment. Data are representative of three independent experiments and error bars represent s.d. of technical replicates (mean±s.d. ), n =3, in a , e . Full size image ERAP1 rescues MHC class I expression in p53-deficient cells To definitively show that MHC I levels in these cells are controlled specifically via the p53–ERAP1 interaction, we employed a ‘knockdown and reinstate’ approach. Two p53-specific small interfering RNA (siRNA) oligos (si-p53-1 and si-p53-2) targeting different mRNA regions of p53 were used to effectively repress p53 expression in HCT116 ( p53 +/+ ) cells, which resulted in a corresponding 50–60% reduction in ERAP1 mRNA ( Fig. 5a ) and protein ( Fig. 5b ) levels. Surface MHC class I expression was also visibly diminished in the p53-knocked down cells compared with cells transfected with negative control siRNA ( Fig. 5c,d ), confirming that endogenous cellular p53 is a potent modifier of MHC class I expression. We repeated this experiment in U2OS ( p53 +/+ ) cells, with comparable results both in terms of downregulated ERAP1 expression following p53 knockdown ( Supplementary Fig. S3a ) and reduced surface MHC class I levels ( Supplementary Fig. S3b–d ). 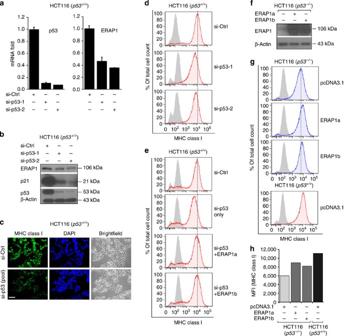Figure 5: Restoration of ERAP1 expression rescues the MHC class I expression. (a) Effect of p53-specific siRNAs in decreasing p53 and ERAP1 mRNA in HCT116 (p53+/+) cells as measured by real-time qPCR. Data are representative of three independent experiments (mean±s.d.). (b) Western blot analysis of ERAP1, p53, p21 and β-actin (loading control) expression in control siRNA (si-Ctrl) or p53 siRNAs (si-p53-1, si-p53-2) transfected HCT116 (p53+/+) cells at 48 h post transfection. (c) Immunofluorescence images of MHC class I expression shown by W6/32 staining in control siRNA (si-Ctrl) or pooled p53 siRNAs (si-p53) transfected HCT116 (p53+/+) cells at 48 h post transfection. DAPI and Brightfield images confirm the relatively equal number of cells captured. Scale bar, 50 μm. (d) Flow cytometric analysis of MHC class I (W6/32 staining) expression in control siRNA (si-Ctrl) or p53 siRNA (si-p53-1, si-p53-2) treated HCT116 (p53+/+) (red) cells at 48 h post treatment. Cells incubated with fluorescence-labelled secondary antibodies alone served as background controls (Grey). Dotted line marked the MFI (mean fluorescence intensity, calculated by FlowJo) of W6/32 signal observed for si-Ctrl-treated cells. (e) Flow cytometric analysis of MHC class I (W6/32 staining) expression when pooled p53 siRNAs (si-p53) were co-transfected with expression plasmids expressing ERAP1a or ERAP1b isoforms into HCT116 (p53+/+) cells. pcDNA3.1 control plasmid was used to balance the total amount of transfected DNA. (f) Expression of overexpressed ERAP1a or ERAP1b proteins in HCT116 (p53−/−) cells as shown by western blot. (g) Flow cytometric analysis of MHC class I (W6/32 staining) expression in ERAP1a or ERAP1b overexpressed HCT116 (p53−/−) (blue) cells. Dotted line marked the MFI of W6/32 signal observed for pcDNA3.1 plasmid control-transfected HCT116 (p53−/−) cells. The pcDNA3.1 control plasmid transfected HCT116 (p53+/+) (red) cells were also analysed for MHC class I expression. The calculated MFI values for all different treatments are shown in (h). Figure 5: Restoration of ERAP1 expression rescues the MHC class I expression. ( a ) Effect of p53-specific siRNAs in decreasing p53 and ERAP1 mRNA in HCT116 ( p53 +/+ ) cells as measured by real-time qPCR. Data are representative of three independent experiments (mean±s.d.). ( b ) Western blot analysis of ERAP1, p53, p21 and β-actin (loading control) expression in control siRNA (si-Ctrl) or p53 siRNAs (si-p53-1, si-p53-2) transfected HCT116 ( p53 +/+ ) cells at 48 h post transfection. ( c ) Immunofluorescence images of MHC class I expression shown by W6/32 staining in control siRNA (si-Ctrl) or pooled p53 siRNAs (si-p53) transfected HCT116 ( p53 +/+ ) cells at 48 h post transfection. DAPI and Brightfield images confirm the relatively equal number of cells captured. Scale bar, 50 μm. ( d ) Flow cytometric analysis of MHC class I (W6/32 staining) expression in control siRNA (si-Ctrl) or p53 siRNA (si-p53-1, si-p53-2) treated HCT116 ( p53 +/+ ) (red) cells at 48 h post treatment. Cells incubated with fluorescence-labelled secondary antibodies alone served as background controls (Grey). Dotted line marked the MFI (mean fluorescence intensity, calculated by FlowJo) of W6/32 signal observed for si-Ctrl-treated cells. ( e ) Flow cytometric analysis of MHC class I (W6/32 staining) expression when pooled p53 siRNAs (si-p53) were co-transfected with expression plasmids expressing ERAP1a or ERAP1b isoforms into HCT116 ( p53 +/+ ) cells. pcDNA3.1 control plasmid was used to balance the total amount of transfected DNA. ( f ) Expression of overexpressed ERAP1a or ERAP1b proteins in HCT116 ( p53 −/− ) cells as shown by western blot. ( g ) Flow cytometric analysis of MHC class I (W6/32 staining) expression in ERAP1a or ERAP1b overexpressed HCT116 ( p53 −/− ) (blue) cells. Dotted line marked the MFI of W6/32 signal observed for pcDNA3.1 plasmid control-transfected HCT116 ( p53 −/− ) cells. The pcDNA3.1 control plasmid transfected HCT116 ( p53 +/+ ) (red) cells were also analysed for MHC class I expression. The calculated MFI values for all different treatments are shown in ( h ). Full size image To further confirm the requirement for ERAP1 in p53-regulated MHC class I expression, we cloned two naturally occurring isoforms of ERAP1 , ERAP1a and ERAP1b, into the pcDNA3.1 expression vector and transfected these functionally similar expression constructs into p53-knocked down cells, to restore ERAP1 expression. HCT116 ( p53 +/+ ) cells were co-transfected with pooled p53 siRNAs (si-p53-1 and si-p53-2, 20 nM each) and ERAP1a or ERAP1b expression constructs. Both combinatorial transfectants exhibited restored MHC class I expression levels as compared with cells transfected with p53 siRNAs alone ( Fig. 5e ). As the p53 +/+ cell lines have a generally higher expression level of ERAP1 than their p53 −/− counterparts ( Fig. 3c ; Supplementary Fig. S4a ), we transfected the ERAP1 constructs into p53 −/− HCT116 and Saos-2 cells to understand whether ERAP1 overexpression ( Fig. 5f ; Supplementary Fig. S4b ) would similarly rescue the MHC class I expression level. Interestingly, expression of either ERAP1a or ERAP1b resulted in a ~1.5–2-fold increase in the expression of MHC class I molecules ( Fig. 5g,h ; Supplementary Fig. S4c,d ). To provide further evidence that MHC class I expression is indeed regulated via p53-mediated ERAP1 activation, we also overexpressed wild-type p53 and this resulted in increased ERAP1 mRNA level ( Supplementary Fig. S5a ) and a significant enhancement of MHC class I expression, but no change was observed in p53 mutant R175H-transfected cells ( Supplementary Fig. S5b,c ). H1N1 PR8-activated p53 upregulates MHC class I expression As a classical tumour suppressor, p53 protects cells against varied stresses, including those caused by viral infection. Influenza A virus was reported to increase p53 activity after infection [19] and thus represents an interesting model pathogen to study p53-regulated pathways. We used the H1N1 PR8 strain to infect a human pulmonary type II epithelial cell line A549, which harbours wild-type p53 (ref. 20 ) and was reported to be highly susceptible to many strains of influenza A virus [19] . A549 cells were inoculated with PR8 at different multiplicities of infection (MOI) (0.5, 1.0 and 2.0) and successful infection confirmed by the presence of cytopathic effect ( Supplementary Fig. S6a ) as well as the expression of viral genes encoding NS1 (non-structural protein 1) and HA (hemagglutinin) ( Supplementary Fig. S6b,c ). The cells infected at MOI 2.0 were collected at 18, 24 or 48 h post infection for measurement of MHC class I expression by flow cytometry. Interestingly, a substantial increase in MHC class I expression was observed as early as 18 h post infection, compared with mock control-treated cells, and the increase was sustained through to the 24 and 48 h time points ( Fig. 6a ). Consistent with previous reports [19] , we observed increased levels of p53 protein in infected cell cultures, much of which was activated, as seen by detection of Ser15-phosphorylated p53 molecules, in contrast to uninfected cell cultures ( Fig. 6b ). We proceeded to ask whether the upregulation of p53 directly contributed to increased MHC class I expression after H1N1 infection. Cells collected at 48 h post virus infection were seeded into chamber slides for simultaneous antibody labelling for MHC class I and p53. Both p53 and MHC class I expression was largely induced in H1N1 PR8-infected cells when compared with mock control. In addition, cells with elevated expression of MHC class I also co-expressed high levels of p53, as seen in the overlay images ( Fig. 6c ). Co-labelling of phospho-Ser15 p53 and MHC I also revealed substantial co-localization ( Fig. 6d ). Similar to the p53 +/+ HCT116 cells, knocking down endogenous p53 using siRNAs ( Fig. 6e ) again resulted in a decrease in MHC class I surface expression in A549 cells ( Fig. 6f,g ). Co-transfection of the wild-type p53 expression plasmid and p53 siRNA restored cellular p53 expression ( Fig. 6e ) and largely rescued the MHC class I expression level ( Fig. 6f,g ), further supporting the direct role of p53 in regulating MHC class I in response to H1N1 infection. Finally, co-labelling the viral NS1 protein together with p53 or phosphorylated p53 (Ser15) showed that infected cells generally upregulated p53 and phosphor-p53 ( Supplementary Fig. S6d,e ), confirming the relationship between virus infection and p53 activation. 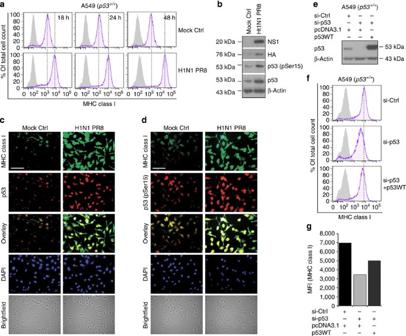Figure 6: Influenza A virus infection-activated p53 enhances MHC class I expression in A549 (p53+/+) cells. (a) Time point flow cytometry analysis of MHC class I expression (W6/32 staining) of H1N1 PR8 (MOI 2.0) or mock control-infected A549 (p53+/+) (purple) cells. Cells incubated with fluorescence-labelled secondary antibodies alone served as background controls (grey). (b) Western blot analysis of PR8 NS1, PR8 HA (hemagglutinin), p53, phosphor-p53 (Ser15) and β-actin (loading control) protein expression at 18 hpi in mock control and H1N1 PR8-infected cells. (c) Immunofluorescence microscopic images of p53 and MHC class I (W6/32) expression in mock control and H1N1 PR8-infected cells at 48 hpi. Overlay images showed co-localization/co-expression of p53 and MHC class I. (d) Immunofluorescence microscopic images of phosphor-p53 (Ser15) and MHC class I (W6/32) expression in mock control and H1N1 PR8-infected cells at 48 hpi. Overlay images showed co-localization/co-expression of phosphor-p53 (Ser15) and MHC class I. DAPI and Brightfield images confirm the relatively equal number of cells captured. Scale bar, 50 μm. (e) Western blot analysis of p53 and β-actin (loading control) protein expression at 48 h in the p53 siRNA-transfected or p53 siRNA (40 nM) and wild-type p53 expression plasmid (3 μg per well) co-transfected A549 (p53+/+) cells. (f) Flow cytometry analysis of MHC class I expression (W6/32 staining) of the p53 siRNA transfected or p53 siRNA and wild-type p53 expression plasmid co-transfected A549 (p53+/+) cells. Dotted line marked the MFI of W6/32 signal observed for control siRNA (si-Ctrl) transfected A549 (p53+/+) cells. The calculated MFI values for all different treatments are shown in (g). Figure 6: Influenza A virus infection-activated p53 enhances MHC class I expression in A549 ( p53 +/+ ) cells. ( a ) Time point flow cytometry analysis of MHC class I expression (W6/32 staining) of H1N1 PR8 (MOI 2.0) or mock control-infected A549 ( p53 +/+ ) (purple) cells. Cells incubated with fluorescence-labelled secondary antibodies alone served as background controls (grey). ( b ) Western blot analysis of PR8 NS1, PR8 HA (hemagglutinin), p53, phosphor-p53 (Ser15) and β-actin (loading control) protein expression at 18 hpi in mock control and H1N1 PR8-infected cells. ( c ) Immunofluorescence microscopic images of p53 and MHC class I (W6/32) expression in mock control and H1N1 PR8-infected cells at 48 hpi. Overlay images showed co-localization/co-expression of p53 and MHC class I. ( d ) Immunofluorescence microscopic images of phosphor-p53 (Ser15) and MHC class I (W6/32) expression in mock control and H1N1 PR8-infected cells at 48 hpi. Overlay images showed co-localization/co-expression of phosphor-p53 (Ser15) and MHC class I. DAPI and Brightfield images confirm the relatively equal number of cells captured. Scale bar, 50 μm. ( e ) Western blot analysis of p53 and β-actin (loading control) protein expression at 48 h in the p53 siRNA-transfected or p53 siRNA (40 nM) and wild-type p53 expression plasmid (3 μg per well) co-transfected A549 ( p53 +/+ ) cells. ( f ) Flow cytometry analysis of MHC class I expression (W6/32 staining) of the p53 siRNA transfected or p53 siRNA and wild-type p53 expression plasmid co-transfected A549 ( p53 +/+ ) cells. Dotted line marked the MFI of W6/32 signal observed for control siRNA (si-Ctrl) transfected A549 ( p53 +/+ ) cells. The calculated MFI values for all different treatments are shown in ( g ). Full size image It is known that viral infection of cells can cause the release of interferons, which in turn will stimulate the upregulation of MHC class I [21] . To determine the contribution of interferons in the infection of A549 cells with PR8, we collected supernatant from infected cells at various time points to measure the release of type I and type II IFNs. The results showed that only IFNβ but not IFNγ is detected in the supernatant of infected A549 cells ( Supplementary Fig. S7a,b ). Neutralization of IFNβ using specific antibodies showed that MHC class I expression can be reduced, although even at the saturation concentration of 10 μg ml −1 of IFNβ antibody, there remains significant level of upregulated MHC class I ( Supplementary Fig. S7c,d ). This suggests that IFNβ alone does not account for the entire effect of PR8-induced MHC class I increase. PR8 enhances MHC I expression via ERAP1 and p53 To establish the role of ERAP1 in the relationship between H1N1 and p53-enhanced MHC class I expression, we first measured mRNA and protein expression of ERAP1 after influenza infection. 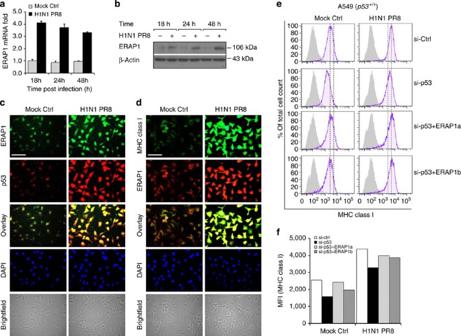Figure 7: Influenza A virus infection enhances MHC class I expression via p53-activated ERAP1 in A549 (p53+/+) cells. (a) Real-time qPCR analysis of ERAP1 mRNA expression in mock control and H1N1 PR8-infected cells. Data are representative of three independent experiments (mean±s.d.). (b) Western blot of ERAP1 and β-actin (loading control) protein expression at different time points in mock control and H1N1 PR8-infected cells. (c) Immunofluorescence microscopic images of p53 and ERAP1 expression in mock control and H1N1 PR8-infected cells at 48 hpi. Overlay images show co-localization/co-expression of p53 and ERAP1. (d) Immunofluorescence microscopic images of ERAP1 and MHC class I (W6/32) expression in mock control and H1N1 PR8-infected cells at 48 hpi. Overlay images showed co-localization/co-expression of ERAP1 and MHC class I. DAPI and Brightfield images confirm the relatively equal number of cells captured. Scale bar, 50 μm. (e) Flow cytometric analysis of MHC class I (W6/32) expression in p53 siRNA transfected or p53 siRNA and ERAP1 expression plasmid (ERAP1a or ERAP1b, 3 μg per well) co-transfected A549 (p53+/+) cells. Twenty four hours after transfection, cells were infected with H1N1 PR8 (MOI 0.5) or mock control and incubated for another 24 h. Dotted lines marked the MFI of W6/32 signal observed for control siRNA (si-Ctrl) transfected A549 (p53+/+) cells in the presence (PR8) or absence (mock control) of virus infection. The calculated MFI values for all different treatments are shown in (f). Figure 7a clearly showed that ERAP1 mRNA expression was upregulated in PR8-infected cells compared with mock-treated cultures. Upregulated ERAP1 protein expression was detected in PR8-infected cells as early as 18 h post infection and continued to accumulate throughout the 48 h ( Fig. 7b ). Next, ERAP1 was visualized alongside MHC I or p53 by fluorescence microscopy; intense ERAP1 labelling was seen in H1N1 PR8-infected cells and this high expression was correlated with increased p53 protein ( Fig. 7c ) and elevated MHC class I expression ( Fig. 7d ). ERAP1 expression was also seen in H1N1 NS1-expressing cells ( Supplementary Fig. S6f ), which was consistent with the observation that p53 and phospho-p53 exhibited co-expression with NS1 ( Supplementary Fig. S6d,e ). To provide further evidence for the proposed pathway of MHC I regulation, p53 siRNAs and ERAP1 expression constructs were again employed. First, A549 cells were reverse transfected with different combinations of p53 siRNAs and ERAP1 constructs and infected with the H1N1 PR8 strain at a low MOI of 0.5 (selected due to the fragility of cells after reverse transfection). The flow cytometric analysis clearly showed that p53 siRNA markedly diminished MHC class I expression in both mock-treated and PR8-infected cells ( Fig. 7e,f ). Cells co-transfected with p53 siRNA and ERAP1a or ERAP1b constructs exhibited similar levels of MHC class I increase as control siRNA-transfected cells after PR8 infection, showing that both ERAP1 isoforms could rescue the low-MHC I phenotype seen in the absence of p53. These observations demonstrated that influenza virus activated p53 which upregulated MHC class I expression via ERAP1, as we observed in the tumour cell lines. Figure 7: Influenza A virus infection enhances MHC class I expression via p53-activated ERAP1 in A549 ( p53 +/+ ) cells. ( a ) Real-time qPCR analysis of ERAP1 mRNA expression in mock control and H1N1 PR8-infected cells. Data are representative of three independent experiments (mean±s.d.). ( b ) Western blot of ERAP1 and β-actin (loading control) protein expression at different time points in mock control and H1N1 PR8-infected cells. ( c ) Immunofluorescence microscopic images of p53 and ERAP1 expression in mock control and H1N1 PR8-infected cells at 48 hpi. Overlay images show co-localization/co-expression of p53 and ERAP1. ( d ) Immunofluorescence microscopic images of ERAP1 and MHC class I (W6/32) expression in mock control and H1N1 PR8-infected cells at 48 hpi. Overlay images showed co-localization/co-expression of ERAP1 and MHC class I. DAPI and Brightfield images confirm the relatively equal number of cells captured. Scale bar, 50 μm. ( e ) Flow cytometric analysis of MHC class I (W6/32) expression in p53 siRNA transfected or p53 siRNA and ERAP1 expression plasmid (ERAP1a or ERAP1b, 3 μg per well) co-transfected A549 ( p53 +/+ ) cells. Twenty four hours after transfection, cells were infected with H1N1 PR8 (MOI 0.5) or mock control and incubated for another 24 h. Dotted lines marked the MFI of W6/32 signal observed for control siRNA (si-Ctrl) transfected A549 ( p53 +/+ ) cells in the presence (PR8) or absence (mock control) of virus infection. The calculated MFI values for all different treatments are shown in ( f ). Full size image In this study, we showed that MHC class I is differentially expressed in p53 +/+ and p53 −/− tumour cell lines. Screening for possible p53-responsive genes that might mediate this effect identified ERAP1 as a potential target. We went on to demonstrate that p53 could directly activate ERAP1 mRNA transcription, and subsequent protein expression, via a bona fide p53RE located in the intron region. Modifying the cellular level of p53 using Nutlin 3 or p53-specific siRNAs led to corresponding changes in ERAP1 and MHC class I expression. We also provided evidence for the relevance of this relationship in the setting of influenza A virus infection, during which p53 was rapidly activated, ERAP1 was upregulated and consequently MHC class I expression was increased. Hence, our findings identified a previously-unknown association between p53 and MHC class I expression, and provided convincing evidence that p53 has a more diverse role than previously recognized. Antigen processing and presentation by MHC class I molecules is critical for immune surveillance. Defects in MHC class I antigen presentation are a common means for cancer cells to evade T-cell recognition [6] . Endoplasmic reticulum aminopeptidase 1 ( ERAP1 ) functions in processing and final trimming of peptides to mature epitopes for loading onto the MHC class I molecules, which is a critical step in completing the MHC class I processing pathway [22] , [23] . Although there are a number of different mechanisms that contribute to MHC loss in tumour cells, the role of p53 as a regulator of MHC expression has not been fully explored. Downregulation of ERAP1 expression was reported in some, but not all, leukemia/lymphoma, carcinoma and melanoma cell lines [13] ; however, the association between ERAP1 and p53 status of the cells in that study was not established. Interestingly, cell lines carrying wild-type p53, such as MCF7 and A549, expressed comparable levels of ERAP1 to EBV-transformed B cells and control cells [13] . This is consistent with our observation of higher ERAP1 protein levels in p53 +/+ HCT116 cells and also suggests that p53 may have a role in regulating ERAP1 expression across a wider range of cell types than tested here. We also reported that p53-inducing agents such as Nutlin 3 and the genotoxic drug 5-FU can activate both ERAP1 and MHC class I expression in a p53-dependent manner in vitro , which is consistent with, and may provide a mechanism for, the observations in a previous study showing that 5-FU treatment of colon and breast carcinoma cell lines increases tumour cell susceptibility to cytotoxic T lymphocyte-mediated lysis [24] . Similar to transformed cells, one of the strategies employed by pathogens to avoid detection and destruction by the host immune system is to downregulate MHC class I expression, as seen during infection with HIV [25] and HBV [26] . Recent evidence showed that ERAP1 is also targeted directly by human cytomegalovirus microRNA miR-US4-1 (ref. 27 ), further indicating the functional importance of ERAP1 in immune surveillance. Influenza A virus infection was previously reported to increase both expression and activity of p53 in p53 +/+ cells such as A549 (ref. 19 ), and thus was used in the current study to extend our observation of p53-regulated MHC class I expression via ERAP1 into pathological conditions of viral infection. We similarly found that PR8-activated p53 in A549 cells, and revealed that this induced elevated MHC class I expression ( Fig. 6a ), which was accompanied by a substantial upregulation of ERAP1 protein ( Fig. 7b ). Co-localization and co-expression of MHC class I, p53 and ERAP1 were also revealed by immunofluorescence microscopy. Although it is known that virus infection induces interferon response and could contribute to MHC class I increase, we showed that blocking of IFNβ using specific antibodies only partially reduces the upregulation of MHC class I in PR8-infected A549 cells ( Supplementary Fig. S7 ), suggesting that factors other than interferon have a role in PR8-induced MHC class I expression. An intriguing study using the human prostate cancer cell line DU145 (ref. 28 ), which harbours a temperature-sensitive mutant allele of p53 that does not function properly at 37 °C (ref. 29 ), revealed that MHC class I expression remained unchanged after influenza A virus infection. When considered alongside our results, this lends further support to the critical role of p53 in regulating MHC I expression via ERAP1 during influenza virus infection. The importance of ERAP1 in MHC class I antigen processing and presentation has been confirmed in vivo by independent studies [8] , [9] , [30] , [31] , and the functional association of ERAP1 expression and the susceptibility of infected cells to virus-specific cytotoxic T lymphocytes (CTLs) had also been previously shown [27] . Together these suggest that p53 may also have a role in the CTL response to infectious diseases such as influenza regulating MHC class I expression through ERAP1. Our data therefore provide a basis for further investigation into the contribution of p53 and its physiological involvement in immunosurveillance. In conclusion, our study clearly establishes the mechanism by which p53 modulates MHC class I expression via regulating ERAP1 and further validates this observation using a viral infection model. Our data, therefore, expand the understanding of the functions of p53 and demonstrates its role in the immune response. Cell lines and cell culture The human colon cancer cell line HCT116 and its derived isogenic p53 −/− cells were kindly provided by Dr. Bert Vogelstein (Johns Hopkins University). The human osteosarcoma cell lines Saos-2 and U2OS were a gift from Dr. Qiang Yu (Genome Institute of Singapore). The human lung carcinoma cell line A549 was purchased from ATCC (CCL-185). All cells were maintained in DMEM supplemented with 10% fetal bovine serum and cultured at 37 °C incubator. Constructs and drugs The p53WT (pCMV-p53) and mutant p53 (pCMV-p53-R175H) expression vectors were provided by Dr. Bert Vogelstein. Expression vectors of five different p53 mutants (C176F, G245D, R273C, R280T and R282W) were generated using QuickChange Site-Directed Mutagenesis Kit (Stratagene) with primer sequences listed in Supplementary Table S1 . Stealth select RNAi duplex for human TP53 gene (si-p53-1: HSS110905, 5′-GCUUCGAGAUGUUCCGAGAGCUGAA-3′; si-p53-2: HSS186390, 5′-GAGUGGAAGGAAAUUUGCGUGUGGA-3′) and negative control siRNA duplex (medium GC) were purchased from Life Technologies. The ORF fragments of ERAP1a or ERAP1b were first isolated from HCT116 ( p53 +/+ ) cells by PCR and then cloned into pcDNA3.1 (+) plasmid (Life Technologies) via In-Fusion Cloning System (Clontech). Primers used are listed in Supplementary Table S2 . Transient transfection of either expression plasmids or siRNAs was mediated by Lipofectamine 2000 reagents (Life Technologies). Nutlin-3 and 5-FU were purchased from Sigma-Aldrich and reconstituted in DMSO. Virus and virus inoculation Human Influenza A virus (H1N1/A/Puerto Rico/8/34) was kindly provided by Dr Vincent Chow (National University of Singapore). Original A549 cells were seeded and after overnight incubation, washed with PBS twice and then infected with influenza virus at a MOI of 0.5, 1.0 or 2.0. After 1 h adsorption, the inocula were removed and the cells were maintained in maintenance media (DMEM containing 25 mM HEPES and 1% BSA) for the indicated time points. To block secreted IFNβ, maintenance media containing different concentrations (0, 1, 5, 10 μg ml −1 ) of neutralizing antibody to IFNβ (FL-187, sc-20107, Santa Cruz Biotechnology) was added to the mock control or H1N1 PR8-infected A549 cells 1 h after virus inoculation and cultured for another 24 h before collection for flow cytometric analysis. Enzyme-linked immunosorbent assay (ELISA) Supernatant of culture medium from H1N1 PR8 or mock control-infected A549 ( p53 +/+ ) cells at different time points was collected by centrifugation for detecting IFNγ and IFNβ production, respectively, by a Human IFNγ ELISA Kit (Thermo Scientific) and a Verikine Human IFN-β ELISA Kit (PBL Interferon Source) according to the manufacturers’ instructions. Concentration of IFNγ or IFNβ release was calculated using standard curve. RNA isolation and real-time qPCR analysis Total RNA from experimental cells was isolated by RNeasy Mini Kit (Qiagen) and cDNA was synthesized by Maxima First Strand cDNA Synthesis Kit (Fermentas). mRNA expression of different genes was analysed by real-time quantitative RT–PCR using KAPA SYBR FAST qPCR Kit (KAPA). HPRT was used as a housekeeping gene with primer set HPRT-F: 5′-GTAATGACCAGTCAACAGGGGAC-3′ and HPRT-R: 5′-CCAGCAAGCTTGCGACCTTGACCA-3′. All other primers for real-time qPCR are listed in Supplementary Table S3 . Western blot Cells were lysed with 1% Nonidet P-40 cell lysis buffer supplemented with the complete protease inhibitor cocktail (Roche) for 30 min at 4 °C and the protein concentration determined by Bradford Protein Assay (Bio-rad). Approximately 20 μg of cell lysate was separated by 7.5–12.5% SDS–PAGE, and transferred to Hybond PVDF membranes (GE Healthcare). Antibodies against p53 (DO-1, sc-126, 1:3,000), p-p53 (Ser15, sc-101762, 1:100), p21 (C-19, sc-397, 1:250), NS1 (NS1-23-1, sc-130568, 1:100), HA (F-7, sc-7392, 1:100) (Santa Cruz Biotechnology), ERAP1 (ab124669, 1:2,000) and ERAP2 (ab69037,1:3,000) (Abcam) were used for protein detection. Equal loading of protein samples was verified with an antibody to β-actin (1:10,000, Millipore). Immunoreactive signals were visualized with enhanced chemiluminescence reagents (GE Healthcare). Full-length images of immunoblots are shown in Supplementary Fig. S8 . Flow cytometry Cells were harvested after different treatments by trypsinization using 0.05% Trypsin-EDTA (Life Technologies) and washed with PBS. Cells were resuspended in labelling buffer (PBS supplemented with 10% FBS and 1% NaN 3 ) to a final concentration of 1 × 10 6 per ml and stained with W6/32 monoclonal antibody (1:10, ATCC: HB-95) or L243 monoclonal antibody (1:10, ATCC: HB-55) at 4 °C for 1 h, followed by donkey-anti-mouse-AF488 secondary antibody (1:400, A21202, Life Technologies) at 4 °C for 30 min. Cells were washed after each incubation and resuspended in 1 ml of labelling buffer for flow cytometric analysis using a LSRII 4-laser flow cytometer (Becton Dickinson). The results were analysed and MFI calculated by FlowJo. Fluorescence microscopy Isogenic HCT116 cells, U2OS and Saos-2 cells underwent different treatments were replated into chamber slides (Becton Dickinson) for overnight culture. Cells were fixed in para-formaldehyde (4% in PBS) at room temperature for 10 min, permeabilized in Triton-X100 (0.1% in PBS) for 3 min and blocked in bovine serum albumin (1% in PBS) for 1 h before incubating with antibodies specific for MHC class I (mouse monoclonal W6/32, 1:10 dilution) then donkey-anti-mouse-AF488 secondary antibody (1:400 dilution, A21202, Life Technologies). Cells were washed with PBS containing 0.1% Tween-20 after each incubation and finally mounted with ProLong Gold antifade reagent with DAPI (Life Technologies). The fluorescence signals were observed and captured using an Axiovert 200 inverted fluorescence microscope (Carl Zeiss). A549 cells infected with H1N1 PR8 or mock control were also seeded, fixed, permeabilized and co-labelled with different combinations of antibodies including mouse monoclonal W6/32 (1:10), goat polyclonal anti-p53 (C-19, sc1311, 1:250 dilution, Santa Cruz Biotechnology), rabbit polyclonal anti-p-p53 (Ser15) (sc-101762, 1:250 dilution, Santa Cruz Biotechnology), rabbit monoclonal anti-ERAP1 (ab124669, 1: 500 dilution, Abcam), and mouse monoclonal anti-NS1 (sc-130568, 1:200 dilution, Santa Cruz Biotechnology) followed by secondary antibodies at 1:400 dilution including donkey-anti-mouse-AF488 (A21202), donkey-anti-goat-AF555 (A21432), goat-anti-rabbit-AF488 (A11034) and goat-anti-rabbit-AF546 (A11035) (Life Technologies). Luciferase assay All luciferase constructs based on LASP1 promoter region used to study the function of p53 mutants and the luciferase construct containing the p21 promoter regions used as positive control have been described previously [16] . To validate the functionality of the proposed response elements of ERAP1, the identified RE sequences were repeated 2–3 times and annealed to be directly cloned between Sac I and Xho I restriction site upstream of the minimal SV40 promoter in pGL3-Promoter vector (Promega). Annealing primers are listed in Supplementary Table S4 . Different promoter luciferase reporter constructs (2 μg ml −1 ) were co-transfected with pCMV-p53, pCMV-p53-mutant or pcDNA3.1 control plasmid (200 ng ml −1 ), together with 20 ng ml −1 of Renilla control vector into HCT116 ( p53 −/− ) cells seeded in 96-well plates. The luciferase activity was measured 30 h post transfection by the Dual-Luciferase Reporter Assay System (Promega). For all luciferase assays, the normalized luciferase activity of each construct (Firefly/Renilla ratio) in the pCMV-p53 or pCMV-p53-mutant co-transfected cells was then compared with that of the pcDNA3.1 control co-transfected cells. ProLabel Protein–DNA binding assay To measure the binding affinity of p53 to the p53-target RE sequence, we performed ProLabel Protein–DNA Binding Assay (Clontech) according to manufacturer’s protocol. The p53WT or different p53 mutants lacking TAD (residue 75-393) was cloned between the Eco R I and Bam H I restriction sites of pProLabel-C vector using universal primer set p53-ProLabel-F: 5′-AAAGAATTCTCCTGCACCAGCAGCTCCTACAC-3′ (forward) and p53-ProLabel-R: 5′-AAAGGATCCTCAGTCTGAGTCAGGCCCTTCTGT-3′ (reverse). The probe sequences used were wild-type p53RE from p21 (Biotin; 5′-GAACATGTCCCAACATGTTG-3′) and ERAP1 (Biotin; 5′-TGTCATGTGTcagGCACATGTTA-3′), as well as mutant p53RE from p21 (Biotin; 5′-GAAAATATCCCAAAATATTG-3′) and ERAP1 (Biotin; 5′-TGTAATATGTcagGCAAATATTA-3′). Whole-genome Exon Array analysis p53WT, the 6 p53 mutant expression vectors and the pcDNA3.1 control plasmid were separately transfected into HCT116 ( p53 −/− ) cells. Total RNA was extracted 24 h post transfection. Total RNA (1 μg) was used as initial material for GeneChip Human Exon 1.0 ST Arrays (Affymetrix) according to manufacturer’s instructions. After washing and staining of hybridized arrays with an Affymetrix Fluidics Station, they were scanned on Gene Array Scanner 2500 (Affymetrix) to capture the raw probe signal intensities in CEL files. Background subtraction, quantile normalization and summarizing probe sets from Affymetrix expression microarrays raw CEL files were done with Affymetrix Power Tools (APT) software. The resulting probeset signals were annotated with Affymetrix annotation library HuEx-1_0-st-v2.na30.hg19.probeset.csv. ChIP-seq and data analysis ChIP using fresh PBMCs extracted from a healthy donor and then treated with 5-FU (50 μg ml −1 ) for 24 h was carried out as described by Wei et al. [32] Approximately 10 ng of ChIP or input DNA was used for library construction and single-end 36 bp sequencing with Illumina Genome Analyser II performed by Genotypic Technology (India) according to standard protocol. Raw illumina ChIP-seq fastq files were analysed at Galaxy ( http://main.g2.bx.psu.edu ) and Galaxy/Cistrome ( http://cistrome.org ). Briefly, single-end ChIP-seq reads were mapped to the human reference genome assembly HG19 using an ultrafast and memory-efficient short read aligner Bowtie [33] taking into account a maximum number of two mismatches permitted in the seed of 28 nt in length. ChIP-seq peak calling from mapped reads via MACS [34] empirically models the sequenced ChIP fragments (tag size of 36 nt) with a dynamic Poisson distribution to effectively capture local biases in the genome sequence, and uses it to improve the spatial resolution of predicted binding sites that satisfied P -value cutoff of 0.00001. R script was used for annotation. Statistical analyses All experiments were repeated at least three times with similar results achieved. Representative images or data are shown. Differences between averages and percentages between control and tests were statistically analysed using paired two-tailed Student’s t -tests. P- values less than 0.05 were considered statistically significant. Accession codes: Microarray data have been deposited in the GEO repository under accession code GSE49046. ChIP-seq data have been deposited in NCBI SRA under accession code SRP027583 . How to cite this article: Wang, B. et al. p53 increases MHC class I expression by upregulating the endoplasmic reticulum aminopeptidase ERAP1. Nat. Commun. 4:2359 doi: 10.1038/ncomms3359 (2013).